High-throughput and combinatorial gene expression on a chip for metabolism-induced toxicology screening Differential expression of various drug-metabolizing enzymes (DMEs) in the human liver may cause deviations of pharmacokinetic profiles, resulting in interindividual variability of drug toxicity and/or efficacy. Here, we present the ‘Transfected Enzyme and Metabolism Chip’ (TeamChip), which predicts potential metabolism-induced drug or drug-candidate toxicity. The TeamChip is prepared by delivering genes into miniaturized three-dimensional cellular microarrays on a micropillar chip using recombinant adenoviruses in a complementary microwell chip. The device enables users to manipulate the expression of individual and multiple human metabolizing-enzyme genes (such as CYP3A4, CYP2D6, CYP2C9, CYP1A2, CYP2E1 and UGT1A4) in THLE-2 cell microarrays. To identify specific enzymes involved in drug detoxification, we created 84 combinations of metabolic-gene expressions in a combinatorial fashion on a single microarray. Thus, the TeamChip platform can provide critical information necessary for evaluating metabolism-induced toxicity in a high-throughput manner. The human body, primarily the liver, contains a variety of oxidative and conjugative enzymes that are involved in the metabolism of the myriad compounds that comprise today’s pharmaceuticals [1] . In many cases, drugs are converted into toxic metabolites by Phase I enzymes, such as the cytochromes P450 (CYP450s), and/or detoxified by Phase II enzymes, such as UDP-glucuronosyltransferases (UGTs) and glutathione S -transferases [2] . Different segments of the population express various levels of drug-metabolizing enzymes because of genetic polymorphisms [3] ; thus, understanding the role of these polymorphic enzymes in drug metabolism is a primary goal of ongoing research and has important implications for future drug development and toxicology testing [4] . In recent years, high-throughput in vitro cell-based assays have emerged to provide insights into drug metabolism and toxicity for various cell lines, including primary hepatocytes and immortalized liver cells expressing CYP450s [5] . Primary hepatocytes, which provide a complete set of drug-metabolizing pathways, have been used extensively for in vitro drug testing, and indeed, have become routine in drug metabolism studies [6] . Nevertheless, primary hepatocytes are expensive and difficult to obtain in large quantities with uniform cell function for high-throughput toxicity screening [7] . Even more problematic is the rapid loss of liver specific functions coupled with variable expression levels of drug-metabolizing enzymes when the cells are maintained under standard in vitro cell culture conditions over time [8] . In addition, primary hepatocytes show high donor variability in terms of drug metabolism, which often results in irreproducible results and significant lab-to-lab variability. For these reasons, immortalized liver cell lines stably expressing a single metabolizing enzyme, as well as non-metabolizing parental cell lines, are often used early in drug discovery to predict the potential for clinical acute hepatotoxicity [9] , [10] and to elucidate roles of specific CYP450s in drug metabolism and metabolic profiling. For example, liver cell lines expressing CYP2C9, CYP2C19 or CYP2D6 have been used to study clinically relevant polymorphisms that may contribute to toxicity [9] . The construction of stable liver cell lines that express multiple drug-metabolizing enzymes is difficult, laborious and time-consuming due to low chromosomal integration frequency and the need for antibiotic selection procedures. Several groups have employed stable transduction methods in recombinant lentivirus microarrays in gelatin coupled with 2D cell monolayers [11] , as well as transient transfection (for example, via lipofectamine-based DNA delivery in microarrays) [12] , albeit with a focus on loss-of-function analyses with interfering RNAs or overexpression of fluorescent proteins. Such 2D, on-chip, gene transduction protocols typically require high titres of recombinant viruses (~10 9 pfu ml −1 ), which pose a safety concern to research personnel, and often lead to difficulty in controlling multiple-gene expression levels without cross-contamination among neighbouring spots on a microarray. Cell detachment from monolayers as a result of a toxic response is also a frequent occurrence. To address these limitations, in the present work we have developed a ‘Transfected Enzyme and Metabolism Chip’ (or TeamChip) that is built upon a robust microarray platform comprising human cell culture and gene transduction with recombinant adenoviruses that carry genes for drug-metabolizing enzymes. We have constructed recombinant adenoviruses and transfected genes encoding multiple drug-metabolizing enzymes into human liver cell lines encapsulated in a hydrogel matrix in 3D (as small as 60 nl). As a result, individual and combinatorial gene transductions have been performed to identify potential toxic responses of model compounds due to drug metabolism. Chip fabrication The TeamChip is based on a complementary arrangement of micropillar and microwell structures prepared by plastic injection molding, which is ideal for mammalian cell culture, enzymatic reactions, viral transduction and high-throughput screening ( Fig. 1 ). The micropillar chip is comprised of poly(styrene- co -maleic anhydride) (PS-MA) and contains 532 micropillars (0.75 mm pillar diameter and 1.5 mm pillar-to-pillar distance) and through-holes between micropillars, which prevent water condensation during incubation. PS-MA provides a reactive functionality for covalent attachment of amine-reactive polymers, such as poly- L -lysine or collagen, ultimately allowing alginate or matrigel spots to attach strongly onto the micropillar surface. Human cells, at controllable seeding densities, are incorporated into the alginate or matrigel 3D matrices. A complementary microwell chip, comprised of polystyrene, has 532 microwells (1.2 mm well diameter and 1.5 mm well-to-well distance) and microbumps between microwells to avoid direct contact with the micropillar chip when the two chips are stamped together. By inserting (stamping) the micropillar into the microwell chip, the cells in the former contact the growth medium in the latter, enabling cell culture to be performed for toxicity studies (typically lasting 2–3 days). The stamped chips are stored in a gas-permeable incubation chamber with water in the periphery of the chamber, preventing spot drying and ensuring effective gas exchange over the entire chip for robust cell culture ( Supplementary Fig. 1 ). 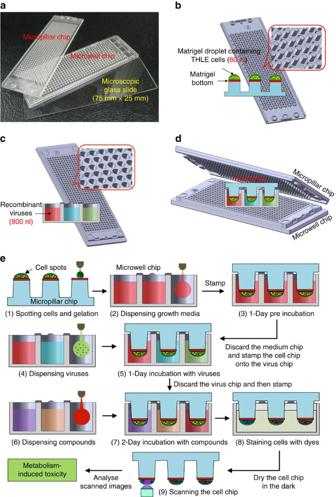Figure 1: TeamChip schematics and photographs. (a) Micropillar/microwell chip components in relation to a standard glass microscope slide. (b) The micropillar chip containing THLE-2 cells encapsulated in matrigel droplets. (c) The microwell chip containing recombinant adenoviruses carrying genes for drug-metabolizing enzymes (the red colour indicates the no-virus control and the two colours represent different viruses). (d) Stamping of the micropillar/microwell chips for drug-metabolizing gene expression. (e) Experimental procedure for use of the TeamChip. Figure 1: TeamChip schematics and photographs. ( a ) Micropillar/microwell chip components in relation to a standard glass microscope slide. ( b ) The micropillar chip containing THLE-2 cells encapsulated in matrigel droplets. ( c ) The microwell chip containing recombinant adenoviruses carrying genes for drug-metabolizing enzymes (the red colour indicates the no-virus control and the two colours represent different viruses). ( d ) Stamping of the micropillar/microwell chips for drug-metabolizing gene expression. ( e ) Experimental procedure for use of the TeamChip. Full size image Individual and multiple-gene transduction on the chip Preliminary experiments were performed, including the optimization of matrices for cell encapsulation that would facilitate high adenoviral gene transduction ( Supplementary Figs 2 and 3 ), the identification of an optimal liver cell line for adenoviral expression of metabolizing enzyme genes ( Supplementary Fig. 4 ), and evaluation of the basal toxicity of recombinant adenoviruses to the optimal liver cell line selected ( Supplementary Fig. 5 ). As a result of these experiments, we focused the TeamChip on THLE-2 cells encapsulated in matrigel and limited the multiplicity of infection (MOI) of recombinant adenoviruses to less than 20. THLE-2 cells are closely related to human hepatocytes [13] , yet have insignificant levels of phase I and II drug-metabolizing enzyme activities, and hence are not expected to produce any basal enzyme interference from the cell line. In addition, basal expression levels of membrane transporters that pump drugs across cellular barriers, are relatively low in THLE-2 cells when compared with HepG2, Hep3B, SK-Hep-1, Huh7 and human hepatocytes [14] . Thus, THLE-2 cells were chosen for the current study. The viral transduction of metabolizing enzyme genes on the TeamChip was performed by spotting 60 nl of THLE-2 cell suspension in matrigel (approximately 180 cells per spot) onto the matrigel-coated micropillar chip. This was followed by gelation for 30 min at 37 °C in an air-tight sealed chamber with eight wells at the bottom containing 0.5 ml of water in each well to prevent spot drying. After preincubation with 800 nl of bronchial epithelial cell growth medium (BEGM) in the complementary microwell chip for 24 h to maintain high cell viability, the THLE-2 cells encapsulated in the matrigel spots on the micropillar chip were then immersed by stamping for 24 h into the microwell chip containing 800 nl of BEGM growth medium with recombinant viruses ( Fig. 1e ). Using a mixture of Ad-GFP and Ad-RFP at different MOIs in the microwell chip, we were able to control the co-expression levels of GFP and RFP in THLE-2 cells on the TeamChip without cross-contamination among neighbouring spots, and the efficiency of viral transduction was as high as 100% after 24 h incubation ( Fig. 2a ). The GFP expression level increased as the concentrations of Ad-GFP increased, whereas the RFP expression level decreased proportionately when Ad-RFP decreased. The average expression levels of GFP and RFP (pg per cell) in each THLE-2 cell were determined from on-chip GFP/RFP calibration curves as a function of the MOI. These results indicate that the levels of either one or two proteins could be controlled on the chip by simply varying the MOIs of recombinant adenoviruses carrying genes for target proteins. 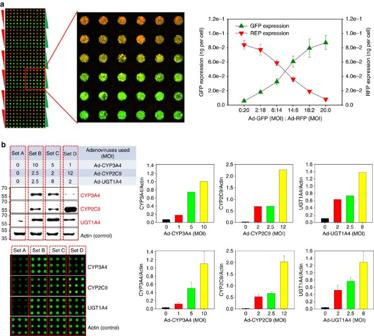Figure 2: Controlled expression of proteins in THLE-2 cells on the TeamChip. (a) Scanned image of the TeamChip containing THLE-2 cells co-expressing GFP and RFP (left) and the expression levels of GFP and RFP in THLE-2 cells achieved by co-transfecting different ratios of adenoviruses carrying genes for GFP (Ad-GFP) and RFP (Ad-RFP; right). (b) Controlled expression of three drug-metabolizing enzymes (CYP3A4, CYP2C9 and UGT1A4) by co-transfecting different ratios of Ad-CYP3A4, Ad-CYP2C9 and Ad-UGT1A4: (top left) western blot analysis of THLE-2 cell monolayers co-expressing CYP3A4, CYP2C9 and UGT1A4 and (bottom left) In-cell immunofluorescence assay of THLE-2 cells co-expressing CYP3A4, CYP2C9 and UGT1A4 on the chip. Three combinations of MOIs of the three recombinant adenoviruses at a total MOI of 15 (sets B, C and D) were used to compare the co-expression levels of the three drug-metabolizing enzymes expressed in THLE-2 cells on the TeamChip with those obtained from THLE-2 cell monolayers in six-well plates. The bar graphs represent the co-expression levels of the three drug-metabolizing enzymes expressed in THLE-2 cell monolayers (top) and THLE-2 cells on the chip (bottom). Figure 2: Controlled expression of proteins in THLE-2 cells on the TeamChip. ( a ) Scanned image of the TeamChip containing THLE-2 cells co-expressing GFP and RFP (left) and the expression levels of GFP and RFP in THLE-2 cells achieved by co-transfecting different ratios of adenoviruses carrying genes for GFP (Ad-GFP) and RFP (Ad-RFP; right). ( b ) Controlled expression of three drug-metabolizing enzymes (CYP3A4, CYP2C9 and UGT1A4) by co-transfecting different ratios of Ad-CYP3A4, Ad-CYP2C9 and Ad-UGT1A4: (top left) western blot analysis of THLE-2 cell monolayers co-expressing CYP3A4, CYP2C9 and UGT1A4 and (bottom left) In-cell immunofluorescence assay of THLE-2 cells co-expressing CYP3A4, CYP2C9 and UGT1A4 on the chip. Three combinations of MOIs of the three recombinant adenoviruses at a total MOI of 15 (sets B, C and D) were used to compare the co-expression levels of the three drug-metabolizing enzymes expressed in THLE-2 cells on the TeamChip with those obtained from THLE-2 cell monolayers in six-well plates. The bar graphs represent the co-expression levels of the three drug-metabolizing enzymes expressed in THLE-2 cell monolayers (top) and THLE-2 cells on the chip (bottom). Full size image With these encouraging results, we proceeded to investigate the expression levels of single CYP450 (CYP2C9) as well as multiple drug-metabolizing enzymes (CYP3A4, CYP2C9 and UGT1A4) in THLE-2 cells on the TeamChip, and for comparison, on monolayers of THLE-2 cells in six-well plates, at varying concentrations of recombinant adenoviruses. As expected, the expression levels of CYP2C9 in THLE-2 cells increased as a function of the MOI of Ad-CYP2C9 added, as determined by in-cell, on-chip immunofluorescence assays. A similar trend was observed for Western blots from THLE-2 cell monolayers in six-well plates ( Supplementary Fig. 6 ). The co-expression levels of CYP3A4, CYP2C9 and UGT1A4 in THLE-2 cells were investigated with mixtures of Ad-CYP3A4, Ad-CYP2C9 and Ad-UGT1A4 at different ratios. We selected three combinations of MOIs of the three recombinant adenoviruses for a total MOI of 15 (for example, 10 MOI+2.5 MOI+2.5 MOI, 5 MOI+2 MOI+8 MOI, and 1 MOI+12 MOI+2 MOI for Ad-CYP3A4, Ad-CYP2C9 and Ad-UGT1A4, respectively), and the expressed metabolizing enzymes in THLE-2 cells were normalized by actin levels to accurately calculate the expression level as a function of cell seeding density. As a result, the co-expression levels of each enzyme in THLE-2 cells on the TeamChip, as well as in the monolayers of THLE-2 cells in six-well plates, were controllable by varying the MOIs of recombinant adenoviruses carrying genes for the drug-metabolizing enzymes ( Fig. 2b ). In addition, the expression levels of the three drug-metabolizing enzymes obtained from THLE-2 cells on the chip were almost identical to those from THLE-2 cell monolayers in six-well plates. Interestingly, CYP2C9 expression in THLE-2 cells at 12 MOI was approximately twofold higher than CYP3A4 expression at 10 MOI, indicating that protein expression levels are highly dependent on the gene being expressed. Although the maximum expression level of each enzyme varied, expression of an individual enzyme could be controlled up to a maximum level by modulating the MOI of the Ad-Enzyme construct. All drug-metabolizing enzymes expressed in THLE-2 cells were reactive against traditional luminescent or fluorogenic substrates ( Supplementary Fig. 7 ), and THLE-2 cells transduced with 10 MOI each of Ad-CYP1A2, CYP2C9 and CYP3A4 gave similar enzyme activities to the respective activities of human hepatocytes ( Supplementary Table 1 ). These results indicate that it is possible to precisely control the expression levels of single or multiple drug-metabolizing enzymes on the TeamChip by varying the ratios of recombinant adenoviruses, which is crucial for the platform’s use as a tool for high-throughput gene transduction. TeamChip expressing single and multiple human DMEs To emulate metabolism of the human liver, four sets of TeamChips were prepared, each set containing four different recombinant adenoviruses added into four horizontal regions of the microwell chip (single virus type or a mixture of virus types per region and four regions per chip) ( Supplementary Table 2 ). These chip experiments were performed with quadruplicate chips ( n =4), and each chip contained triplicate cell spots. Six model hepatotoxic compounds (acetaminophen, bromfenac, flutamide, tamoxifen, trifluoperazine and troglitazone) were dispensed into six vertical blocks on the additional microwell chip (one compound with six dosages within each 12 × 6 mini-array block and six blocks per chip) ( Supplementary Table 2 ). The six compounds selected have elicited warnings for hepatotoxicity due to adverse drug reactions in vivo or have been withdrawn from the market entirely because of idiosyncratic hepatotoxicity. The micropillar chips containing 60 nl of THLE-2 cell spots were stamped onto the microwell chips containing 720 nl of four different recombinant adenoviruses in BEGM medium for 24 h, followed by stamping of the micropillar chips containing infected THLE-2 cells into fresh microwell chips containing 800 nl of six compounds in BEGM medium for 48 h for metabolism-induced toxicity assays ( Fig. 1e ). Thus, 24 dose-response curves consisting of six doses (triplicate microwells per dose) were obtained from a single TeamChip. For virus set no. 1 ( Supplementary Table 2 ), the toxicities of the six compounds were compared with those of their metabolites generated by CYP2C9, CYP2D6, CYP3A4 and CYP1A2 in THLE-2 cells on the TeamChip infected by Ad-CYP2C9, Ad-CYP2D6, Ad-CYP3A4 and Ad-CYP1A2, respectively, each at 15 MOI ( Fig. 3a ). IC 50 values were obtained and analysis of variance (ANOVA) was performed to identify statistically significant differences between the non-expressed enzyme control and expressed enzyme test conditions. It should be noted that the quadruplicate chip results reported here were performed on different days, that is, n =4. 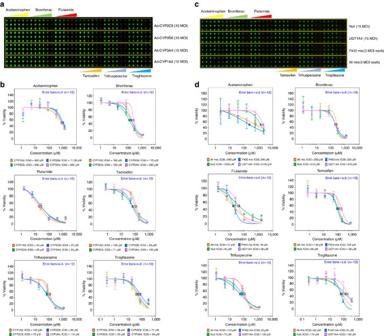Figure 3: Effects of human DMEs expressed in THLE-2 cells on the toxicity of model compounds. (a) Toxicity of six test compounds against THLE-2 cells expressing single drug-metabolizing enzymes on the TeamChip: scanned image of the chip containing THLE-2 cells exposed to adenoviruses and compounds. (b) Dose-response curves for the six compounds (n=3, replicated 4 times). (c) Toxicity of six test compounds against THLE-2 cells expressing multiple drug-metabolizing enzymes on the chip: scanned image of the chip containing THLE-2 cells exposed to adenoviruses and compounds. (d) Dose-response curves for the six compounds (n=3, replicated four times). UGT1A4, P450 Mix and All Mix were expressed in THLE-2 cells on the chip by exposing Ad-UGT1A4 (15 MOI), Ad-P450 Mix (3 MOI each) and Ad-All Mix (3 MOI each). Adenovirus carrying CMV promoter alone (Ad-Null, no drug-metabolizing enzyme expressed) was used as a parent compound-alone control. Figure 3: Effects of human DMEs expressed in THLE-2 cells on the toxicity of model compounds. ( a ) Toxicity of six test compounds against THLE-2 cells expressing single drug-metabolizing enzymes on the TeamChip: scanned image of the chip containing THLE-2 cells exposed to adenoviruses and compounds. ( b ) Dose-response curves for the six compounds ( n =3, replicated 4 times). ( c ) Toxicity of six test compounds against THLE-2 cells expressing multiple drug-metabolizing enzymes on the chip: scanned image of the chip containing THLE-2 cells exposed to adenoviruses and compounds. ( d ) Dose-response curves for the six compounds ( n =3, replicated four times). UGT1A4, P450 Mix and All Mix were expressed in THLE-2 cells on the chip by exposing Ad-UGT1A4 (15 MOI), Ad-P450 Mix (3 MOI each) and Ad-All Mix (3 MOI each). Adenovirus carrying CMV promoter alone (Ad-Null, no drug-metabolizing enzyme expressed) was used as a parent compound-alone control. Full size image As summarized in Table 1 , the toxicity of the analgesic/antipyretic acetaminophen against THLE-2 cells was enhanced by transduction with Ad-CYP2C9 ( P <0.05; one-way ANOVA), Ad-CYP3A4 ( P <0.05; one-way ANOVA) and Ad-CYP1A2 ( P <0.01; one-way ANOVA), but not with Ad-CYP2D6. In addition, statistical difference was evident between Ad-CYP1A2 versus CYP2D6 ( P <0.05; one-way ANOVA). Enhanced toxicity versus the no-enzyme control was also obtained for the Ad-P450 Mix (a mixture of Ad-CYP1A2, Ad-CYP3A4, Ad-CYP2C9, Ad-CYP2D6 and Ad-CYP2E1 at 3 MOI of each virus), or Ad-All Mix (a mixture of Ad-P450 Mix and Ad-UGT1A4 at 3 MOI of each virus). Conversely, acetaminophen toxicity against THLE-2 cells was reduced following transduction by Ad-UGT1A4. These results indicate that CYP450 isoforms and UGT1A4 play an important role in enhanced toxicity and detoxification of acetaminophen, respectively. Acetaminophen is oxidized by CYP450 catalysis, generating a reactive metabolite, N -acetyl- p -benzoquinone imine (NAPQI), which is hepatotoxic, depletes glutathione (GSH), resulting in covalent binding of NAPQI to cellular proteins [15] , and is proposed to be a major cause of liver failure [16] , [17] . It is well known that CYP2E1, CYP3A4, CYP1A2 are the most relevant P450s for the generation of the toxic metabolites of acetaminophen [18] , [19] , although CYP2D6 may be important but only at high (>2 mM) doses of acetaminophen [20] . Table 1 IC 50 values (μM) of six test compounds obtained from the TeamChip. Full size table Interestingly, the influence of CYP2E1 is readily apparent from the P450 Mix and All Mix data for acetaminophen ( Table 1 ). The IC 50 values for both the P450 Mix and the All Mix are significantly lower than the IC 50 values of any of the four individual CYP450 isoforms. The key difference among these sets of experiments is the presence of the CYP2E1 in the expressed enzyme mixtures, as this isoform is well known to be involved in acetaminophen metabolism [18] . Indeed, a dose response for the 15 MOI Ad-CYP2E1 ( Supplementary Fig. 8 ) yields an IC 50 =180±50 μM (footnote to Table 1 ). To study mechanism-based toxicity of acetaminophen, we investigated the effects of ketoconazole (CYP3A4 inhibitor) and buthionine sulfoximine (BSO, an inhibitor of gamma-glutamylcysteine synthetase, and hence an inhibitor of GSH synthesis) in the TeamChip with THLE-2 cells expressing CYP3A4 ( Fig. 4a,b and Supplementary Table 3 ). Intracellular levels of GSH were measured for CYP3A4-expressing THLE-2 cells on the TeamChip in the presence and absence of ketoconazole and BSO ( Fig. 4c,d ). The viability of CYP3A4-expressing THLE-2 cells exposed to BSO significantly decreased, whereas the viability of THLE-2 cells exposed to ketoconazole was only minimally influenced by CYP3A4 expression ( Fig. 4a and Supplementary Table 3 ). Cell viability, therefore, was clearly related to the depletion of intracellular GSH ( Fig. 4c,d ). Moreover, as a result of CYP3A4 inhibition, the intracellular GSH concentrations in CYP3A4-expressing THLE-2 cells exposed to ketoconazole were unchanged at varying concentrations of acetaminophen. Conversely, the intracellular GSH concentrations in THLE-2 cells exposed to BSO were approximately twofold lower than those of the THLE-2 cell controls as a result of inhibition of GSH synthesis by BSO ( Fig. 4c,d ). These results suggest that the enhanced toxicity of acetaminophen on CYP3A4-expressing THLE-2 cells exposed to BSO was due to the lack of sufficient GSH available to detoxify the reactive intermediate, NAPQI. To further confirm the protective mechanism of GSH in acetaminophen metabolism, we measured via liquid chromatography–mass spectrometry the formation of the GSH conjugate with NAPQI in CYP3A4-expressing THLE-2 cells ( Supplementary Fig. 9 ) [21] . 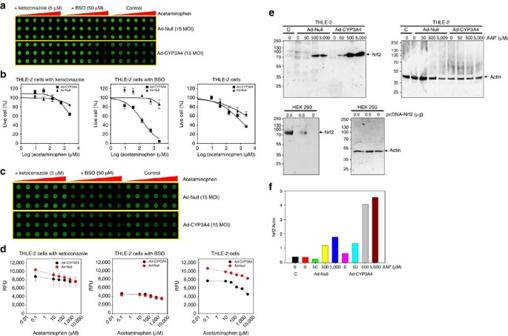Figure 4: Effects of ketoconazole and BSO on CYP3A4-expressing THLE-2 cells on the TeamChip. (a) Toxicity of acetaminophen against THLE-2 cells expressing CYP3A4 on the chip: (top) scanned image of the chip containing THLE-2 cells (control, 15 MOI of Ad-Null) and THLE-2 cells expressing CYP3A4 (15 MOI of Ad-CYP3A4) exposed to 5 μM of ketoconazole as well as 50 μM of BSO in the presence of varying concentrations of acetaminophen for 48 h. (b) Dose-response curves for acetaminophen under different conditions (n=3). The corresponding IC50values are summarized inSupplementary Table 4. (c) GSH content in THLE-2 cells on the TeamChip: scanned image of the chip after staining with a thiol green dye in the intracellular GSH assay kit. (d) Quantitative analysis of GSH levels in THLE-2 cells on the TeamChip (n=3). (e) Western blot analysis of nuclear Nrf2 levels in THLE-2 cells exposed to vehicle (0.1% dimethyl sulfoxide) or different concentrations of acetaminophen for 12 h after transduction with Ad-Null or Ad-CYP3A4 (left). Positive control (293 cells expressing Nrf2) and negative control (293 cells with no Nrf2 expression) were used to authenticate Nrf2 expression (bottom). Actin was probed as a loading control (top right). C, control (no viral transduction); AAP, acetaminophen. (f) Bar graph represents densitometric analysis of nuclear Nrf2 content in AAP-treated THLE-2 cells. Figure 4: Effects of ketoconazole and BSO on CYP3A4-expressing THLE-2 cells on the TeamChip. ( a ) Toxicity of acetaminophen against THLE-2 cells expressing CYP3A4 on the chip: (top) scanned image of the chip containing THLE-2 cells (control, 15 MOI of Ad-Null) and THLE-2 cells expressing CYP3A4 (15 MOI of Ad-CYP3A4) exposed to 5 μM of ketoconazole as well as 50 μM of BSO in the presence of varying concentrations of acetaminophen for 48 h. ( b ) Dose-response curves for acetaminophen under different conditions ( n =3). The corresponding IC 50 values are summarized in Supplementary Table 4 . ( c ) GSH content in THLE-2 cells on the TeamChip: scanned image of the chip after staining with a thiol green dye in the intracellular GSH assay kit. ( d ) Quantitative analysis of GSH levels in THLE-2 cells on the TeamChip ( n =3). ( e ) Western blot analysis of nuclear Nrf2 levels in THLE-2 cells exposed to vehicle (0.1% dimethyl sulfoxide) or different concentrations of acetaminophen for 12 h after transduction with Ad-Null or Ad-CYP3A4 (left). Positive control (293 cells expressing Nrf2) and negative control (293 cells with no Nrf2 expression) were used to authenticate Nrf2 expression (bottom). Actin was probed as a loading control (top right). C, control (no viral transduction); AAP, acetaminophen. ( f ) Bar graph represents densitometric analysis of nuclear Nrf2 content in AAP-treated THLE-2 cells. Full size image We also investigated the activation of transcription factor Nrf2, which serves to protect mammalian cells against chemical and oxidative stress. It is known that CYP3A4-generated reactive metabolites of acetaminophen lead to increased levels of Nrf2 (ref. 17 ). The nuclear level of Nrf2 in CYP3A4-expressing THLE-2 cells increased as the acetaminophen concentration increased ( Fig. 4e,f ). These results, in aggregate, indicate that CYP3A4 expression in THLE-2 cells contributed to the increase of reactive metabolites (NAPQI), activating the protective mechanism (Nrf2) in the cell. Thus, the TeamChip can be used to provide mechanistic information on hepatotoxicity [22] caused by CYP450-generated reactive metabolite(s), demonstrated in this case using acetaminophen as an example. The toxicity of the nonsteroidal antiandrogen flutamide against THLE-2 cells was enhanced by transduction with Ad-CYP1A2 ( P <0.05; one-way ANOVA), Ad-P450 Mix ( P <0.05; one-way ANOVA) and Ad-All Mix ( P <0.01; one-way ANOVA). It is well known that flutamide is metabolized by CYP1A2 to 2-hydroxylflutamide. Flutamide and its major metabolite inhibit taurocholate efflux in human hepatocytes, resulting in time- and concentration-dependent toxicity as assessed by inhibition of protein synthesis [23] , [24] , [25] . Such time-dependent toxicity may not be evident in the TeamChip during the time scale of the experiment. The toxicity of the antiestrogen tamoxifen was enhanced on transduction with Ad-CYP2D6 ( P <0.05; one-way ANOVA) and strongly detoxified with transduction by Ad-UGT1A4 ( P <0.01; one-way ANOVA); both outcomes are similar to known tamoxifen metabolism (for example, primarily CYP2D6 and CYP3A4 activation to reactive metabolites that are subsequently inactivated via glucuronidation and sulfation through various UGTs and sulfotransferases) [26] , [27] . It should be noted that in the absence of a relatively strong metabolizing enzyme of tamoxifen (for example, CYP2D6), other enzymes are capable of contributing to tamoxifen oxidation. In particular, CYP2C9 expression in hepatocytes with inactive CYP2D6 indicates a role for the CYP2C9 isoform [28] . Hence, there is a role for both isoforms in tamoxifen metabolism. The antidiabetes drug troglitazone, which was withdrawn from the market due to hepatotoxicity [29] , [30] , showed enhanced toxicity following transduction with Ad-CYP2C9, Ad-CYP3A4, CYP1A2, Ad-P450 Mix and Ad-All Mix, and reduced toxicity with transduction by Ad-UGT1A4. These results are closely correlated with known metabolism profiles of troglitazone [29] . Similar results were obtained from the TeamChip expressing various levels of CYP3A4 and UGT1A4 ( Supplementary Fig. 10 and Supplementary Table 4 ). Minimal shifts in the toxicity profiles of bromfenac and trifluoperazine were observed, which once again, closely correlates with known metabolism profiles of these compounds [31] , [32] . Thus, the TeamChip is able to replicate known metabolism profiles of compounds that undergo metabolism-induced hepatotoxicity mediated by CYP450s, as well as detoxification by UGTs. The CYP-inactive compounds doxorubicin and rotenone were used as negative controls to test their toxicity against THLE-2 cells expressing CYP1A2, CYP2C9, CYP2D6, CYP3A4 and P450 Mix, and to evaluate apoptotic mechanisms in THLE-2 cells [33] ( Supplementary Figs 11 and 12 ). 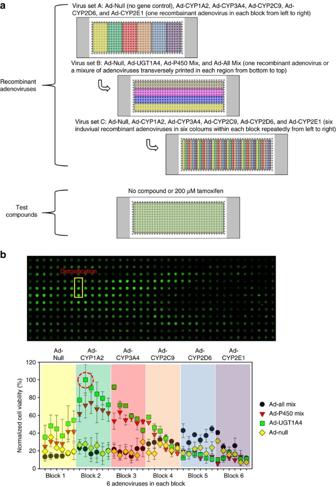Figure 5: Effects of combinatorial expression of human drug-metabolizing enzymes on the toxicity of tamoxifen. (a) Layout of the microwell chip containing 84 combinations of multiple recombinant adenoviruses (three sets of recombinant adenoviruses dispensed sequentially) to prepare the TeamChip for high-throughput gene transduction, and an additional microwell chip containing 200 μM tamoxifen for metabolism-induced toxicity screening. (b) Scanned image of THLE-2 cells expressing 84 combinations of multiple drug-metabolizing enzymes on the chip exposed to 200 μM tamoxifen for 48 h (top) and normalized THLE-2 cell viability at different drug-metabolizing enzyme expression levels (bottom). The viability of multiple drug-metabolizing enzyme-expressing THLE-2 cells exposed to tamoxifen was normalized by the fluorescent intensity of THLE-2 cells incubated in the absence of compound. The least toxic region in the scanned image is highlighted in a yellow box, and the red circle in the graph designates normalized THLE-2 cell viability calculated from the least toxic region. The toxicity of both doxorubicin and rotenone was only minimally affected by the expression of the CYP isoforms in THLE-2 cells, consistent with the expectation that doxorubicin and rotenone are not metabolized by CYPs [34] , [35] ( Supplementary Table 5 ). Moreover, doxorubicin and rotenone increased the number of apoptotic cells in a dose-dependent manner, whereas acetaminophen did not ( Supplementary Figure 12 ). Thus, the hepatotoxicity of doxorubicin and rotenone was linked to apoptosis, whereas the hepatotoxicity of acetaminophen was connected to reactive metabolite-mediated GSH depletion and oxidative stress. Therefore, the TeamChip enabled us to rapidly distinguish mechanisms of hepatotoxicity by various drugs (for example, CYP inhibition, GSH depletion and apoptosis). Combinatorial gene transduction on the TeamChip A key advantage of the TeamChip platform is the ability to combinatorially create various transduction combinations. To achieve 84 combinations of multiple drug-metabolizing enzymes expressed in THLE-2 cells on a single TeamChip, 240 nl of individual recombinant adenoviruses carrying genes for CYP450 enzymes (Ad-CYP1A2, Ad-CYP3A4, Ad-CYP2C9, Ad-CYP2D6, Ad-CYP2E1 and Ad-Null as a control, 15 MOI each, Virus Set A) were dispensed in blocks 1–6. This was followed by dispensing 240 nl of Ad-Null (15 MOI), Ad-UGT1A4 (15 MOI), Ad-P450 Mix (3 MOI each) and Ad-All Mix (3 MOI each), Virus Set B, in four regions transversely, and then dispensing 240 nl of six individual recombinant adenoviruses carrying genes for CYP450 enzymes (15 MOI each), Virus Set C, in six columns within each block repeatedly ( Fig. 5a ). Thus, in each spot, the THLE-2 cells were exposed to anywhere from one adenovirus-containing drug-metabolizing gene up to six adenovirus-containing drug-metabolizing genes. Metabolism-induced toxicity against THLE-2 cells was tested on the TeamChip with these 84 expression combinations of drug-metabolizing enzymes in the presence of 200 μM tamoxifen for 48 h, and the viability of THLE-2 cells exposed to the compound was normalized by the control of TeamChip exposed to BEGM medium (no compound). A tamoxifen dosage higher than its IC 50 value (90 μM) was selected to identify drug-metabolizing enzymes involved in the detoxification of tamoxifen. Thus, THLE-2 cells exposed to 200 μM tamoxifen would show minimal viability unless tamoxifen is detoxified by drug-metabolizing enzymes expressed in THLE-2 cells. Figure 5: Effects of combinatorial expression of human drug-metabolizing enzymes on the toxicity of tamoxifen. ( a ) Layout of the microwell chip containing 84 combinations of multiple recombinant adenoviruses (three sets of recombinant adenoviruses dispensed sequentially) to prepare the TeamChip for high-throughput gene transduction, and an additional microwell chip containing 200 μM tamoxifen for metabolism-induced toxicity screening. ( b ) Scanned image of THLE-2 cells expressing 84 combinations of multiple drug-metabolizing enzymes on the chip exposed to 200 μM tamoxifen for 48 h (top) and normalized THLE-2 cell viability at different drug-metabolizing enzyme expression levels (bottom). The viability of multiple drug-metabolizing enzyme-expressing THLE-2 cells exposed to tamoxifen was normalized by the fluorescent intensity of THLE-2 cells incubated in the absence of compound. The least toxic region in the scanned image is highlighted in a yellow box, and the red circle in the graph designates normalized THLE-2 cell viability calculated from the least toxic region. Full size image The results obtained clearly illustrate the ability of the TeamChip to induce drug-metabolizing activity within transfected cells ( Fig. 5b , Supplementary Table 6 ). Several spots showed increased cell viability after compound incubation with expressed drug-metabolizing enzymes due to detoxification reactions (‘hits’), along with the responsible drug-metabolizing enzymes. Specifically, tamoxifen was substantially detoxified when THLE-2 cells were exposed to a combination of two or three recombinant adenoviruses, such as Ad-CYP1A2 at 10 MOI plus Ad-UGT1A4 at 5 MOI (the highest detoxifying combination) or Ad-CYP1A2 at 5 MOI plus Ad-CYP3A4 at 5 MOI plus Ad-UGT1A4 at 5 MOI (the second highly detoxifying combination), rather than a single adenovirus. These results imply that co-expression of CYP1A2 and UGT1A4, or of CYP1A2, CYP3A4 and UGT1A4 are involved in detoxification mechanisms of tamoxifen. It is well known that tamoxifen is transformed into N -desmethyl-tamoxifen by CYP1A2 and CYP3A4, and tamoxifen and its metabolites are further converted to N -glucuronide or O -glucuronide metabolites by UGT1A4 (refs 26 , 36 ). To investigate specific detoxification pathways of tamoxifen, it will be necessary to scale-up the metabolism reactions and isolate the metabolites for further analysis. The TeamChip platform for high-throughput viral transduction of genes in 3D cell culture microarrays was developed for use in high-throughput, mechanism-based drug metabolism toxicity screening. Intrinsic to this work is the goal of developing a robust high-throughput, three-dimensional (3D) cell-based screening platform for more ‘ in vivo -like’ 3D cell cultures, which can incorporate numerous genetic variations of drug metabolism into toxicology screening. To achieve this goal, we designed and fabricated a robust micropillar/microwell chip, which can employ recombinant adenoviruses carrying genes for drug-metabolizing enzymes. It was possible to control the expression levels of drug-metabolizing enzymes on the chip platform without cross-contamination among neighbouring spots. Recent reports indicated that the IC 50 value of acetaminophen obtained from HepaRG cells in 2D culture was 26.3 mM, whereas those from HepaRG cells in 3D culture was 2.7 mM [37] . This lower IC 50 value appeared to result from higher expression levels of CYP450 isoforms in the 3D HepaRG cultures [37] , [38] , although it may also have been partly due to more in vivo -like cellular behaviour [38] . This result is consistent with the low IC 50 value (~0.8 mM) observed in 3D-cultured THLE-2 cells expressing high CYP3A4 levels on the TeamChip. Therefore, expression levels of CYP450s in cells, and particularly in 3D cultures, is an important variable that can be controlled on the TeamChip to obtain metabolism-mediated toxicity information from test compounds. Existing in vitro cell-based hepatotoxicity screens, including primary hepatocytes, terminally differentiated hepatocytes from stem cells, and liver cell lines stably or transiently expressing each individual drug-metabolizing enzyme, would be useful tools for assessing overall drug metabolism and toxicology. However, each lacks the ability to provide mechanistic insights into adverse drug reactions from specific combinations of multiple drug-metabolizing enzymes because they provide either all drug-metabolizing enzymes (for example, hepatocytes) or a single enzyme (for example, liver cell lines stably expressing a single drug-metabolizing enzyme). Moreover, these systems have limited capability to predict human toxicity for various segments of the population, and they do not enable the necessary throughput for evaluating metabolism-induced toxicity at an early stage of drug discovery. Stable cell lines transfected with cDNAs encoding individual drug-metabolizing enzymes have been developed to assist in identifying precise roles of specific CYP450s in drug metabolism and in investigating drug–drug interactions [39] . For example, THLE-2 cells have been used to construct a stable cell line that expresses consistently high levels of individual human CYP450 enzymes under the control of a cytomegalovirus (CMV) promoter [40] . The expression level and activity of CYP450s in THLE-2 cells were markedly elevated (25–90 fold) when compared with primary human hepatocytes, thus enabling investigation of potential contributions of individual CYP450 isoforms to human toxicity. The limitations of CYP450-expressing stable cell lines, however, include a predictive result limited to a single metabolizing enzyme, difficulty in identifying major metabolic pathways due to having only a single CYP450 isoform involved, poor sensitivity due to the lack of a specific enzyme necessary for metabolism to reactive metabolites, and lack of in vivo relevance [9] . An approach to construct stable liver cell lines that express combinations of two drug-metabolizing enzymes has been reported previously to improve the sensitivity of drug metabolism [41] . However, the construction of stable cell lines that express more than two drug-metabolizing enzymes has been limited due to low chromosomal integration frequency and antibiotic selection procedures [42] , [43] . In contrast, the TeamChip incorporates multiple and controllable variations of drug metabolism into a toxicology screening platform, which is simple to operate. Moreover, by elucidating the effect of given DMEs and their mixtures on drug toxicity, the roles of these enzymes on drug metabolism in vitro can be correlated to in vivo responses. Herein, we demonstrated that the TeamChip, expressing single or multiple drug-metabolizing enzymes or 84 combinations of drug-metabolizing enzymes, could be used to decipher complex mechanisms behind drug metabolism and toxicology. For example, tamoxifen, an important drug for the treatment of oestrogen receptor positive breast cancer that is hepatotoxic at relatively high dosages, is well known to be metabolized by specific drug-metabolizing enzymes. As a result, the therapeutic response to tamoxifen has a high degree of interindividual variability because of its extensive metabolism in vivo [26] . Using the TeamChip, we demonstrated that CYP1A2, CYP3A4 and UGT1A4 are involved in the detoxification processes of tamoxifen, and two/three metabolism reactions are more efficient in tamoxifen detoxification than a single metabolism reaction. The degree of control over drug metabolism afforded by the TeamChip platform creates the opportunity to tailor the TeamChip to different population subgroups, and ultimately to individual patients, by controlling gene expression levels of various drug-metabolizing enzymes in human liver cells to match enzyme levels to those representative of a subgroup or unique to an individual. If successful, this approach can provide critical information needed for the design of stratified or patient-specific treatment regimens, as well as for the identification of pharmacologically safe and effective lead compounds for advancement to clinical trials. Unlike conventional in vitro cell-based hepatotoxicity screens, the TeamChip requires very small amounts of cells, viruses and test compounds for screening, and it is anticipated that the chip platform could be extended to other cell-based in vitro assays. The TeamChip is particularly relevant for mechanistic toxicology, whereby the function of specific human drug-metabolizing enzymes are identified that contribute to the toxicity profile of a given test compound. We anticipate that the TeamChip, on transduction with genes involved in signalling pathways, can also be used to identify positive and negative modulators with gain- and loss-of-function genomic screening. This potential breadth in targets and assays makes the TeamChip a highly flexible platform for drug discovery. Chip fabrication The micropillar microwell chips were manufactured by plastic injection molding using an injection molder (Sodic Plustech, USA). A metal mold was made of carbon steel by using a CNC milling machine (Mage-III, Roku-Roku, Japan). The micropillar chip, made of poly(styrene- co -maleic anhydride) (PS-MA, Polyscope, Netherlands), contains 532 micropillars (0.75 mm micropillar diameter and 1.5 mm pillar-to-pillar distance). The microwell chip, made of polystyrene (LG Chem., South Korea), has 532 complementary microwells (1.2 mm microwell diameter and 1.5 mm well-to-well distance). Both chips are similar in size to conventional glass microscope slides (75 mm × 25 mm). Construction of recombinant adenoviruses Recombinant adenoviruses carrying genes for human drug-metabolizing enzymes (Ad-CYP1A2, Ad-CYP3A4, Ad-CYP2C9, Ad-CYP2D6, Ad-CYP2E1 and Ad-UGT1A4) were constructed from human cDNA library with corresponding primers ( Supplementary Table 7 ) using Adeno-X expression system 3, followed by the manufacture’s protocols (Clontech). Briefly, the PCR products encoding human drug-metabolizing enzymes were purified and subcloned into pAdenoX-CMV using In-Fusion cloning method ( Supplementary Fig. 13 ). The resultant plasmids were transformed into Stellar competent cells, and positive colonies were screened using endonuclease analysis and DNA sequencing to identify the correct recombinant clones. This recombinant adenoviral DNA was then transfected into HEK 293 cells (ATCC, Manassas, VA, USA) for 10 days until the full cytopathic effect was achieved. The cells were harvested and underwent three cycles of freezing and thawing. The cell lysates were then collected after centrifugation. This cell lysate stock, containing primary recombinant adenovirus, was further applied to a series of consecutive propagation procedure for in vitro packaging. The recombinant adenoviruses were amplified by adding the adenoviruses (1–5 MOI) into HEK 293 cells (~70% confluent). Finally, the propagated viral particles were concentrated with a centrifugal filter device (Centricon Plus-70, Millipore) to reduce the volume ~50-fold. The amplified recombinant adenoviruses were titrated by end-point dilution assay (Clontech). The activities of human drug-metabolizing enzymes (CYP1A2, CYP2C9, CYP2D6, CYP3A4, CYP2E1 and UGT1A4) expressed in THLE-2 cells (from ATCC) in 96-well plates were verified by the P450-Glo assay (Promega) for CYP2C9 and CYP3A4, UGT-Glo assay (Promega) for UGT1A4, and Vivid CYP450 assay (Invitrogen) for CYP1A2, CYP2D6 and CYP2E1 ( Supplementary Fig. 7 ). Briefly, THLE-2 cells, seeded into 96-well plates, were treated with 10 MOI of recombinant adenoviruses in BEGM medium (Lonza), and then the medium containing adenoviruses was replaced with the medium containing 50 μM of Luciferin-PFBE (for CYP2C9 and CYP3A4) or 30 μM of proluciferin UGT substrate (for UGT1A4). After incubating for 8 h at 37 °C in a humidified 5% CO 2 incubator (Thermo Scientific), 100 μl of the BEGM medium were added to 100 μl of Luciferin Detection Reagent. After incubating for 20 min at room temperature, the luminescence was measured with a luminometer. In the case of CYP1A2, CYP2D6 and CYP2E1, THLE-2 cells, seeded into 96-well plates, were treated with 10 MOI of recombinant adenoviruses in BEGM medium, and then the medium was replaced with 200 μl of the medium containing 50 μM of Vivid EOMCC. After incubating for 8 h at 37 °C in the 5% CO 2 incubator, the fluorescent intensity in the medium was measured with a microplate reader (SpectraMax M5, Molecular Devices) at excitation 405 nm and emission 460 nm. Human cell culture THLE-2 cells (ATCC) were grown in BEGM medium supplemented with 10% fetal bovine serum (FBS from Sigma-Aldrich), 1% Penicillin–Streptomycin (PS from Invitrogen), and 50 μg ml −1 gentamycin (Sigma-Aldrich) in PureCol/fibronectin-coated T-75 flasks in a humidified 5% CO 2 incubator at 37 °C. The suspensions of THLE-2 cells were prepared by trypsinizing a confluent layer of the cells with 1 ml of 0.05% trypsin-0.53 mM EDTA (Invitrogen) from the culture flask, and resuspending the cells in 7 ml of 10% FBS-supplemented BEGM. After centrifugation at 1,000 r.p.m. for 4 min, the supernatant was removed and the cell pellets were resuspended with 10% FBS-supplemented BEGM to a final concentration of 6 × 10 6 cells per ml. Hep3B, HepG2, Beas-2 and H4IIE cells were cultured according to ATCC’s protocols and cell suspensions were prepared similarly. Preparation of the TeamChip and compound screening To attach cell spots on the surface of micropillars, the micropillar chip was coated with a 1:1 (v/v) mixture of matrigel (BD biosciences) and Dulbecco’s phosphate-buffered saline (DPBS from Gibco) by dipping the tips of micropillars in the matrigel/DPBS solution on ice and then dried at room temperature. The micropillar chip containing THLE-2 cells was prepared by dispensing 60 nl of cold THLE-2 cell suspension in 50% matrigel (to a final seeding density of 3 × 10 6 cells ml −1 ) on top of the dried matrigel/DPBS coating using the microarray spotter, followed by incubating the chip in an air-tightly sealed chamber with water for 30 min at 37 °C. While spotting THLE-2 cells, the micropillar chip was placed on a chilling slide deck at 4 °C to retard evaporation of water in the spots. After matrigel gelation, the micropillar chip was immediately stamped on top of the microwell chip containing 800 nl of BEGM medium by aligning the edges of the chips and then the stamped chip was incubated in the gas-permeable chamber with water in the CO 2 incubator at 37 °C for 18 h before virus transduction. For gene transduction, 720 nl of recombinant adenoviruses in BEGM medium was dispensed in the microwell chip, and then the micropillar chip containing THLE-2 cells was stamped onto the virus-containing microwell chip after discarding the BEGM-containing microwell chip. The stamped chip was placed in the CO 2 incubator at 37 °C for 1 day for the expression of target proteins, followed by discarding the virus-containing microwell chip. The micropillar chip with infected THLE-2 cells (the TeamChip) was then immediately stamped onto the microwell chip containing 800 nl of test compounds in BEGM medium, and the stamped chip was incubated for 2 days for metabolism-induced toxicity assays. At the end of the 2-day incubation period, the TeamChip was washed twice with 6 ml of DPBS for 10 min each and then stained with 2 ml of a Live/Dead staining dye solution (Invitrogen) for 1 h in the dark. The Live/Dead staining dye solution was prepared by adding 1.0 μl of calcein AM (4 mM) and 4.0 μl of ethidium homodimer-1 (2 mM) in 8 ml of DPBS. The stained TeamChip was washed three times with 6 ml of DPBS for 15 min each and then dried completely in the dark. The location of each cell spot, where the compounds were added, was detected by imaging the entire TeamChip using blue laser (488 nm) and standard blue filter for green dye and blue laser and 645AF75/594 filter for red dye in GenePix Professional 4200A scanner (MDS Analytical Technologies). Data files were saved as single tiff images. The spot size in all images was approximately 750 μm in diameter. To produce a conventional sigmoidal dose-response curve, the green fluorescence intensities of all cell spots were normalized to the fluorescence intensity of 100% live cell spots (for example, cell spots contacted with no compound) and then plotted against the logarithm of test compound concentrations. The sigmoidal dose-response curves (variable slope) and IC 50 values for each compound and adenovirus tested were obtained using equation 1: where IC 50 is the midpoint of the curve, H is the hill slope, X is the logarithm of test concentration, and Y is the response (% live cells), starting at bottom and going to top with a sigmoid shape. The IC 50 value represents the concentration of a compound at which cell growth is inhibited by 50%. GSH levels in THLE-2 cells on the TeamChip were quantified by an intracellular GSH assay kit from Abcam. Briefly, the TeamChip was washed twice with 6 ml of DPBS for 10-min periods and then stained with 2 ml of a thiol green dye solution in the GSH assay kit for 20 min in the dark. The stained TeamChip was washed three times with 6 ml of DPBS for 15-min periods and then dried completely in the dark. The thiol green dye solution was prepared by adding 5 μl of 200X thiol green dye in 1 ml of BEGM media. The TeamChip stained with thiol green dye was visualized with the GenePix Professional 4200A scanner at 488 nm excitation (blue laser) and 520 nm emission (standard green filter). Apoptosis of THLE-2 cells on the TeamChip was measured using YO-PRO-1/propidium iodide in Vybrant apoptosis assay kit (Invitrogen). Briefly, all reagents were prepared according to manufacturer’s instructions. Staining and washing were carried out by the aforementioned protocol. The TeamChip was visualized at 488 nm excitation (blue laser) and 530 nm emission (standard green filter)/>575 nm (yellow filter). The apoptotic cells were stained with the green fluorescent YO-PRO-1 dye and the necrotic cells were stained with propidium iodide. Statistical analysis of IC 50 values Statistical analysis was performed with GraphPad Prism 4.0 (GraphPad Software, San Diego, CA) using IC 50 values and standard errors obtained from quadruplicate chips, each chip containing triplicates of cell spots. One-way (ANOVA) was used to compare the mean IC 50 values of test compounds obtained from THLE-2 cells expressing no enzyme (negative control, exposed to Ad-Null) with those from THLE-2 cells expressing human drug-metabolizing enzymes. Statistically significant IC 50 difference between no-enzyme control and enzyme test conditions was indicated as * for P <0.05 and ** for P <0.01. Western blot analysis THLE-2 cell lysates obtained from the monolayers of THLE-2 cells expressing human drug-metabolizing enzymes in six-well plates were subjected to electrophoresis on 10% sodium dodecyl sulfate-polyacrylamide gel electrophoresis and transferred to a nitrocellulose membrane. The membranes were incubated with 8% (w/v) skim milk in phosphate-buffered saline (PBS) containing 0.1% (v/v) Tween 20 (PBS-T) for blocking, and then reacted with specific primary antibodies, such as anti-CYP2C9 (1:500 dilution; Thermo Scientific), anti-CYP3A4 (1:500 dilution; Thermo Scientific), anti-UGT1A4 (1:500 dilution; Sigma), anti-actin antibody (1:1,000 dilution, Sigma) or anti-Nrf2 antibody (1:1,000 dilution, Abcam). Secondary antibodies (1:2,000 dilution; Invitrogen) conjugated with horseradish peroxidase were used and immunoreactive proteins were detected with the enhanced chemiluminescence reagent (Pierce). For Nrf2 nuclear accumulation experiments, around 10 7 cells of THLE-2 cells were lysed after treating with acetaminophen for 12 h. Following treatment of cells, cytosolic and nuclear fractions were prepared using the classical method [44] and stored at −80 °C before analysis. The HEK 293 cells expressing Nrf2 were prepared after transfecting pcDNA-Nrf2 (Addgene) with lipofectamine (Invitrogen) and used as a positive control Nrf2 expression. In-cell immunofluorescence assay on the TeamChip TeamChips were rinsed twice in PBS for 10 min each, followed by fixation with 3.7% formaldehyde in PBS for 20 min at room temperature and permeabilized with 0.1% Triton-X-100 in PBS for 10 min [45] . The chips were rinsed twice in PBS, incubated overnight in a blocking solution (SuperBlock, Pierce), and then rinsed three times in PBS-T for 5 min each. The primary antibodies (anti-CYP2C9, anti-CYP3A4 or anti-UGT1A4 at 1:250 dilution in PBS-T containing 1% (w/v) bovine serum albumin were then added to the TeamChips, and the chips were incubated overnight at 4 °C. The chips were washed three times in PBS-T for 15 min each, and the secondary antibodies (horseradish peroxidase-conjugated goat-anti mouse or rabbit IgG, Invitrogen) at 1:500 dilution in PBS-T containing 1% (w/v) bovine serum albumin were incubated with the TeamChip for 3 h at room temperature. A tyramide signal amplification kit (Invitrogen) was used according to manufacturer’s instructions to detect the human drug-metabolizing enzymes expressed in THLE-2 cells through fluorescence analysis. The scanned images were obtained from the GenePix scanner and analysed by GenePix Pro 6.0. The fluorescent signal from actin was used as an internal control. How to cite this article: Kwon, S. J. et al. High-throughput and combinatorial gene expression on a chip for metabolism-induced toxicology screening. Nat. Commun. 5:3739 doi: 10.1038/ncomms4739 (2014).